Phosphorylation status determines the opposing functions of Smad2/Smad3 as STAT3 cofactors in TH17 differentiation Transforming growth factor-β (TGF-β) and interleukin-6 (IL-6) are the pivotal cytokines to induce IL-17-producing CD4 + T helper cells (T H 17); yet their signalling network remains largely unknown. Here we show that the highly homologous TGF-β receptor-regulated Smads (R-Smads): Smad2 and Smad3 oppositely modify STAT3-induced transcription of IL-17A and retinoic acid receptor-related orphan nuclear receptor, RORγt encoded by Rorc , by acting as a co-activator and co-repressor of STAT3, respectively. Smad2 linker phosphorylated by extracellular signal-regulated kinase (ERK) at the serine 255 residue interacts with STAT3 and p300 to transactivate, whereas carboxy-terminal unphosphorylated Smad3 interacts with STAT3 and protein inhibitor of activated STAT3 (PIAS3) to repress the Rorc and Il17a genes. Our work uncovers carboxy-terminal phosphorylation-independent noncanonical R-Smad–STAT3 signalling network in T H 17 differentiation. Transforming growth factor-β (TGF-β) had been appreciated as the most potent immunosuppressive cytokine, suppressing the differentiation and functions of effector immune cells as inducing suppressor immune cells [1] , [2] . However, since identified as the requisite cytokine in combination with interleukin (IL)-6 for the differentiation of IL-17-producing CD4 + T helper cell (T H 17) through inducing a master transcription factor, retinoic acid-related orphan receptor-γt (RORγt) and IL-17 (refs 3 , 4 ), context-dependent multidirectional roles of TGF-β have been highlighted in immune regulation, similarly to its roles in carcinogenesis and cancer progression [5] . T H 17 is a crucial effector CD4 + T-cell subset in inflammation, protective mechanisms against infections, tumour immunity and autoimmune responses [6] , [7] . Crucial pathogenic role of T H 17 in autoimmune diseases such as rheumatoid arthritis (RA) has been well demonstrated by numerous studies including the pioneer work showing the attenuation of collagen-induced arthritis (CIA) in the mice deficient in IL-17A (ref. 8 ). Intracellular signal transduction of TGF-β superfamily cytokines is initiated by two types of serine/threonine kinase transmembrane receptors [9] , [10] . TGF-β ligands bind to TGF-β type II receptor (TβRII), which transphosphorylates and activates TGF-β type I receptor (TβRI). TGF-β-specific receptor-regulated Smads (R-Smads), Smad2 and Smad3, are composed of N-terminal Mad homology-1 (MH1) domain, linker region and carboxy-terminal (C-terminal) MH2 domain that contains two serine residues phosphorylated by TβRI. Activated TβRI phosphorylates serine residues, SSXS in MH2 domains of R-Smads, which form the heterodimer complex with common-mediator Smad, Smad4, to regulate transcription of the target genes [10] , [11] . TβRI phosphorylates not only the C-termini of R-Smads but also activates various protein kinases including mitogen-activated protein kinases (MAPKs): extracellular signal-regulated kinase (ERK), c-Jun N-terminal kinase (JNK) and p38 MAPK (p38), which then phosphorylate the variable linker regions of R-Smads [11] , [12] , [13] . MAPKs are shared by T-cell receptor (TCR) and various cytokines including IL-6 as the crucial intracellular signalling mediators for effector T-cell differentiation [14] , [15] . IL-6 and other cytokines such as IL-21 and IL-23 that induce and maintain T H 17 activate STAT3, a critical transcription factor for T H 17 differentiation and the pathogenesis of autoimmune diseases including RA [16] . In contrast to the established essential roles of STAT3-mediated IL-6 signalling in T H 17 differentiation, molecular mechanisms by which R-Smads regulate T H 17 differentiation still remain under debate. Despite their high amino-acid sequence homology, Smad2 and Smad3 exert both redundant and distinct functions in TGF-β signalling depending on the context [17] . Several reports have shown contradictory results regarding their roles in T H 17 differentiation: Smad2 as the essential inducer [18] , [19] , Smad3 as the negative regulator [20] , [21] or non-Smad signals as the crucial inducers with irrelevance of R-Smads [22] , [23] . Thus far, roles of canonical TGF-β signalling through C-terminal phosphorylation of R-Smads for T H 17 differentiation have been examined. MAPK signalling pathways, which phosphorylate linker regions of R-Smads, play crucial roles in differentiation and functions of effector T cells [1] , [2] , [24] . However, whether diverse phosphorylation status of R-Smads, such as linker phosphorylation or unphosphorylation, affects T H 17 differentiation remains largely undetermined. In this study, we seek to determine the mechanisms whereby R-Smads regulate T H 17 differentiation. We investigate the molecular mechanisms how Smad2 and Smad3 regulate the transcription of the essential genes for T H 17 and examine the pathophysiological roles of R-Smads in T H 17-related inflammatory disease by applying a CIA model to Smad2-deficient ( Smad2 −/− ), Smad3-deficient ( Smad3 −/− ) and control wild-type mice. We discover the opposing functions of Smad2 and Smad3 as transcription cofactors of STAT3 in T H 17 differentiation independently of Smad4: the canonical partner of C-terminally phosphorylated R-Smads. Mechanistic studies show that the phosphorylation status of R-Smads distinctively modulates STAT3-induced transcription of the Rorc and Il17a genes. Linker-phosphorylated Smad2 (pSmad2L) at the residue Ser255 via ERK serves as a STAT3 co-activator in cooperation with p300, whereas C-terminally unphosphorylated Smad3 (unphosphorylated Smad3C) serves as a STAT3 co-repressor in cooperation with protein inhibitor of activated STAT3 (PIAS3), the negative regulator of STAT3 signalling. Opposing roles of Smad2 and Smad3 in CIA To examine the pathophysiological roles of R-Smads in T H 17-mediated inflammatory disease, we applied a CIA model to T-cell-specific ( Cd4Cre;Smad2 +/+, +/fl, fl/fl ), inducible systemic ( Mx-1Cre;Smad2 +/+, +/fl, fl/fl ) Smad2 conditional knockout mice and Smad3 heterozygote ( Smad3 +/+, +/− ) mice. They showed normal immune phenotypes with C57BL/6 background in a specific pathogen-free environment ( Supplementary Fig. 1 ), indicating that R-Smads are dispensable for immune homeostasis. T-cell-specific and systemic deletion of Smad2 ameliorated, whereas Smad3 heterozygosity exacerbated CIA ( Fig. 1a and Supplementary Fig. 2a ). Because both systemic and T-cell-specific deletion of Smad2 showed the same phenotype ( Supplementary Fig. 2a,b ), we used Cd4Cre;Smad2 +/+,+/fl. fl/fl mice for further study. Cd4Cre;Smad2 fl/fl mice showed significant amelioration in joint lesions, whereas Smad3 +/− mice showed proliferative detritic synovitis with mononuclear cell infiltration and joint destruction ( Fig. 1b , upper). Evaluation of proteoglycan and mucopolysaccharide of cartilage by staining with toluidine blue and Safranin O showed the significant maintenance of cartilages in Cd4Cre;Smad2 fl/fl mice and marked destruction of cartilages in Smad3 +/− mice ( Fig. 1b , lower). Accumulation of CD4 + , RORγt + and IL-17A + cells in the joint lesions was ameliorated in Cd4Cre;Smad2 fl/fl mice, whereas it was exacerbated in Smad3 +/− mice ( Supplementary Figs 3–5 ). Consistent with the joint lesions, IL-17A + , RORγt + , IL-17A + TNF-α + and IL-17A + RORγt + CD4 + T cells decreased in the draining lymph nodes of the arthritic joints of Cd4Cre;Smad2 fl/fl mice and Mx-1Cre;Smad2 fl/fl mice, whereas they increased significantly in those of Smad3 +/− mice ( Fig. 1c and Supplementary Fig. 2a ). Smad genotypes did not affect other effector T-cell subsets, such as IL-6 + CD4 + , TNF-α + CD4 + , T H 1 (T-bet + IFN-γ + CD4 + ), natural and inducible T reg cells (CD103 − Foxp3 + CD4 + , CD103 + Foxp3 + CD4 + ), naive and memory CD4 + (CD44 low CD62L high , CD44 high CD62L low ) and CD8 + (CD44 low , CD44 high ) T cells in the draining lymph nodes of the arthritic joints ( Supplementary Fig. 6 ). Thus, Smad2 and Smad3 have the opposing roles in T H 17 differentiation in the pathogenesis of CIA. 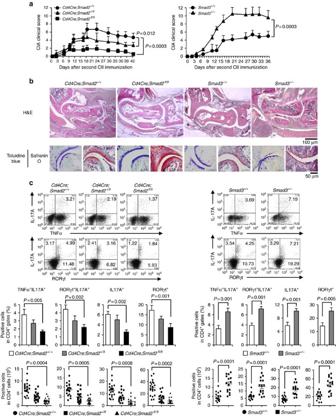Figure 1: Opposing effects of Smad2 and Smad3 on TH17 response in CIA. Cd4Cre;Smad2+/+, +/fl, fl/flandSmad3+/+, +/−mice were immunized with type II collagen emulsified in complete Freund adjuvant twice in 3 weeks interval to induce CIA. (a) CIA scoring courses ofCd4Cre;Smad2+/+,Cd4Cre;Smad2+/fl,Cd4Cre;Smad2fl/flmice (left,n=11/Cd4Cre;Smad2genotype) andSmad3+/+,Smad3+/−mice (right,n=13/Smad3genotype) withPvalues (two-way analysis of variance (ANOVA) test). (b) Pathological analyses of the joint sections (haematoxylin and eosin, H&E, magnification, × 40, scale bar, 100 μm, toluidine blue and safranin O, magnification, × 200, scale bar, 50 μm). (c) Flow cytometry analyses of IL-17A+TNF-α+CD4+T cells and RORγt+IL-17A+CD4+T cells in the draining lymph nodes ofCd4Cre;Smad2+/+,+/fl, fl/fl(n=20/Cd4Cre;Smad2genotype) andSmad3+/+,+/−mice (n=15/Smad3genotype) on day 14 after second immunization. Graphs show the percentages and cell numbers of IL-17A+, RORγt+, IL-17A+TNF-α+and IL-17A+RORγt+in CD4+gates in the draining lymph nodes. Data are from one experiment representative of seven (a,b), four (c,Cd4Cre;Smad2) or three (c,Smad3) independent experiments. Graphs show mean+s.d. withPvalues (unpaired Student’st-test). Figure 1: Opposing effects of Smad2 and Smad3 on T H 17 response in CIA. Cd4Cre;Smad2 +/+, +/fl, fl/fl and Smad3 +/+, +/− mice were immunized with type II collagen emulsified in complete Freund adjuvant twice in 3 weeks interval to induce CIA. ( a ) CIA scoring courses of Cd4Cre;Smad2 +/+ , Cd4Cre;Smad2 +/fl , Cd4Cre;Smad2 fl/fl mice (left, n =11/ Cd4Cre;Smad2 genotype) and Smad3 +/+ , Smad3 +/− mice (right, n =13/ Smad3 genotype) with P values (two-way analysis of variance (ANOVA) test). ( b ) Pathological analyses of the joint sections (haematoxylin and eosin, H&E, magnification, × 40, scale bar, 100 μm, toluidine blue and safranin O, magnification, × 200, scale bar, 50 μm). ( c ) Flow cytometry analyses of IL-17A + TNF-α + CD4 + T cells and RORγt + IL-17A + CD4 + T cells in the draining lymph nodes of Cd4Cre;Smad2 +/+,+/fl, fl/fl ( n =20/ Cd4Cre;Smad2 genotype) and Smad3 +/+,+/− mice ( n =15/ Smad3 genotype) on day 14 after second immunization. Graphs show the percentages and cell numbers of IL-17A + , RORγt + , IL-17A + TNF-α + and IL-17A + RORγt + in CD4 + gates in the draining lymph nodes. Data are from one experiment representative of seven ( a , b ), four ( c , Cd4Cre;Smad2 ) or three ( c , Smad3 ) independent experiments. Graphs show mean+s.d. with P values (unpaired Student’s t -test). Full size image Opposing functions of Smad2 and Smad3 as STAT3 cofactors IL-6 is the main arthritogenic cytokine and TGF-β is produced and activated in the inflammatory lesions [1] , [2] , [25] . Because IL-6 and TGF-β are the pivotal cytokines to induce T H 17 differentiation, we cultured Smad2 −/− or Smad3 −/− CD4 + T cells under T H 17-polarizing condition with IL-6 and TGF-β (ref. 3 ) to examine the mechanisms whereby R-Smads regulate T H 17 differentiation. Expression levels of protein and mRNA of RORγt and IL-17A decreased in Smad2 −/− CD4 + T cells, whereas those increased in Smad3 −/− CD4 + T cells ( Fig. 2a,b ). The mRNA levels of T H 17-inducing genes ( Batf , Il23r , Il6 , Il6ra , Il21 and Il21r ) and T H 17-suppressing genes ( Il2 , Il2ra , Tbet and Eomesodermin ) were unaffected in both Smad2 −/− and Smad3 −/− CD4 + T cells ( Supplementary Fig. 7 ), suggesting that R-Smads regulate T H 17 differentiation by specifically targeting the Rorc and Il17a genes. Because IL-6 or TGF-β alone has little effect on T H 17 differentiation [3] and STAT3-mediated IL-6 signalling is crucial for T H 17 differentiation [16] , we examined whether R-Smads regulate STAT3-induced transcription of RORγt and IL-17A in CD4 + T cells cultured under T H 17-polarizing condition by promoter assays with the luciferase reporters spanning 2 kb upstream of the first exons of the Rorc and Il17a genes ( Fig. 2c ). STAT3 or Smad2 alone induced their promoter activities, whereas Smad3 alone had no effect. Smad2 further enhanced, whereas Smad3 suppressed STAT3-induced reporter activation. Co-transfection of Smad4 with R-Smads and STAT3 did not show the additive effects. We next determined the binding of R-Smads to the proximal promoter regions of the Rorc and Il17a genes in T H 17 cells by chromatin immunoprecipitation (ChIP) using the primers to detect the DNA-binding sequences of Smads and STAT3 (refs 10 , 26 , 27 ). Smad2 and Smad3 were bound to the same sites in the Rorc promoter, whereas they were bound to the distinct sites in the Il17a promoter ( Fig. 2d ). Active promoters are characterized by histone acetylation and trimethylation of H3K4, whereas repressed inactive chromatin is marked by methylation of H3K27 and H3K9 (ref. 28 ). Smad2-binding sites in the Il17a promoter showed higher acetylation of histone H3 and trimethylation of histone H3K4, which correlate with transcriptionally active chromatin ( Supplementary Fig. 8a ). By contrast, Smad3-binding sites in the Il17a promoter showed higher trimethylation of histone H3K27, which correlate with transcriptionally inactive chromatin ( Supplementary Fig. 8b ). These data suggest that Smad2 and Smad3 have the opposing roles in STAT3-induced transcription of the Rorc and Il17a genes. 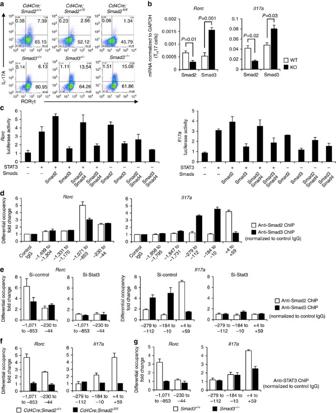Figure 2: Opposing roles of Smad2 and Smad3 in STAT3-induced TH17 differentiation. Purified CD4+T cells were activated under TH17-polarizing condition for 3 days. (a) Flow cytometry analyses of IL-17A and RORγt inSmad2+/+,+/−, −/−andSmad3+/+,+/−, −/−CD4+T cells. (b) Quantitative RT–PCR analysis of theIl17aandRorcmRNA inSmad2+/+, −/−andSmad3+/+, −/−TH17 cells (n=7). (c) Effects of Smads on STAT3-induced activation of theRorcpromoter and theIl17apromoter constructs transfected in TH17 cells were analysed using luciferase assay. (d) Binding of Smad2 and Smad3 to the proximal promoter regions of theRorcgene and theIl17agene in TH17 cells was determined using ChIP. (e) Requirement of STAT3 for the binding of Smad2 and Smad3 to the proximal promoter regions of theRorcgene and theIl17agene was determined with ChIP using STAT3 knockdown TH17 cells. Requirement of Smad2 and Smad3 for the binding of STAT3 to the proximal promoter regions of theRorcgene and theIl17agene was determined with ChIP using (f)Smad2−/−or (g)Smad3−/−TH17 cells. ChIP data are shown as differential occupancy fold changes. Data are from one experiment representative of seven (a,d), three (c), two (e) or five (f,g) independent experiments or pooled from seven experiments (b). Each experiment (a–g) was performed in triplicate (n=3). Data are mean+s.d. or mean+s.d. withPvalues (b, unpaired Student’st-test). Figure 2: Opposing roles of Smad2 and Smad3 in STAT3-induced T H 17 differentiation. Purified CD4 + T cells were activated under T H 17-polarizing condition for 3 days. ( a ) Flow cytometry analyses of IL-17A and RORγt in Smad2 +/+,+/−, −/− and Smad3 +/+,+/−, −/− CD4 + T cells. ( b ) Quantitative RT–PCR analysis of the Il17a and Rorc mRNA in Smad2 +/+, −/− and Smad3 +/+, −/− T H 17 cells ( n =7). ( c ) Effects of Smads on STAT3-induced activation of the Rorc promoter and the Il17a promoter constructs transfected in T H 17 cells were analysed using luciferase assay. ( d ) Binding of Smad2 and Smad3 to the proximal promoter regions of the Rorc gene and the Il17a gene in T H 17 cells was determined using ChIP. ( e ) Requirement of STAT3 for the binding of Smad2 and Smad3 to the proximal promoter regions of the Rorc gene and the Il17a gene was determined with ChIP using STAT3 knockdown T H 17 cells. Requirement of Smad2 and Smad3 for the binding of STAT3 to the proximal promoter regions of the Rorc gene and the Il17a gene was determined with ChIP using ( f ) Smad2 −/− or ( g ) Smad3 −/− T H 17 cells. ChIP data are shown as differential occupancy fold changes. Data are from one experiment representative of seven ( a , d ), three ( c ), two ( e ) or five ( f , g ) independent experiments or pooled from seven experiments ( b ). Each experiment ( a – g ) was performed in triplicate ( n =3). Data are mean+s.d. or mean+s.d. with P values ( b , unpaired Student’s t -test). Full size image We next examined whether STAT3 was necessary for R-Smads to bind to these sites by STAT3 knockdown using short interfering RNA (siRNA) in T H 17 cells ( Supplementary Fig. 9 ). STAT3 knockdown completely abolished the binding of R-Smads to these sites ( Fig. 2e ). We then confirmed whether R-Smads are sufficient for STAT3 to bind to these sites using Smad2 −/− and Smad3 −/− T H 17 cells. STAT3 bound to the Smad2/3-binding sites in the Rorc promoter or the Smad2-binding site in the Il17a promoter ( Fig. 2f,g , white bars). Deficiency of Smad2 or Smad3 prevented STAT3 from binding to these sites ( Fig. 2f,g , black bars). Thus, R-Smads and STAT3 are mutually required to bind to the proximal promoters of the Rorc and Il17a genes. Taken together, Smad2 functions as a transcription co-activator, whereas Smad3 functions as a transcription co-repressor of STAT3 in T H 17 differentiation. Linker-phosphorylated Smad2 induces T H 17 differentiation We investigated the mechanism how Smad2 functions as a transcription co-activator of STAT3. Proximity ligation assays (PLA) confirmed the endogenous close proximity between Smad2 and STAT3 in T H 17 cells ( Fig. 3a , left). We found that pSmad2L had close proximity with STAT3 in T H 17 cells ( Fig. 3a , right). By contrast, C-terminally phosphorylated Smad2 (pSmad2C) did not show close proximity with STAT3 ( Fig. 3a , middle). PLA and immunoprecipitation of 293T cells transfected with the various deletion mutants of Smad2 showed that Smad2 linker deletion mutants (MH1 and MH2) [29] failed to bind with STAT3 ( Fig. 3b and Supplementary Fig. 10a ). Transfection of the linker variants of Smad2 showed that the mutant of the linker serine residue 255 to alanine, Smad2 (S255A) [30] , failed to bind with STAT3 ( Fig. 3c and Supplementary Fig. 10b ). Luciferase reporter assays showed that Smad2 (S255A) failed to enhance STAT3-induced activation of the Rorc and Il17 a promoters ( Fig. 3d ). Overexpression of Smad2 (S255A) in CD4 + T cells cultured under T H 17-polarizing condition impaired T H 17 differentiation ( Fig. 3e ). Therefore, pSmad2L (Ser255) is essential for T H 17 differentiation. 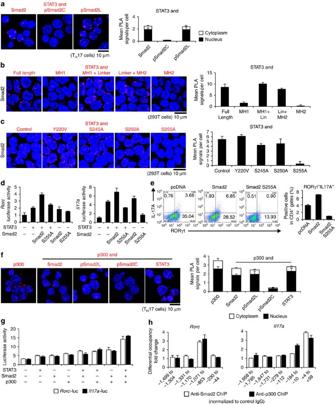Figure 3: Linker-phosphorylated Smad2 (S255)–STAT3–p300 complex transactivates theRorcandIl17a. Interactions of endogenous proteins in TH17 cells and exogenous proteins in 293T cells were determined by PLA. PLA signals (a–c,f) were quantified using the BlobFinder software (scale bars, 10 μm; nucleus, black; cytoplasm, white,n=10 fields). (a) Endogenous interaction between Smad2 and STAT3 in TH17 cells. (b) Effects of truncated mutations in Smad2 on the interaction with STAT3 in 293T cells. (c) Effects of linker domain variations in Smad2 on the interaction with STAT3 in 293T cells. (d) Effects of Smad2 (S255A) on STAT3-induced activation of theRorcpromoter and theIl17apromoter constructs transfected in TH17 cells were analysed by luciferase assay. (e) Flow cytometry analyses of IL-17A+RORγt+CD4+T cells transduced with the indicated DNA constructs using Nucleofector (n=2). (f) Endogenous interactions between p300 and Smad2 or STAT3 in TH17 cells were determined using PLA. (g) Effects of p300 on Smad2/STAT3-induced activation of theRorcpromoter (white) and theIl17apromoter (black) constructs transfected in 293T cells were analysed by luciferase assay. (h) Binding of Smad2 (white) and p300 (black) to the proximal promoter regions of theRorcgene and theIl17agene in TH17 cells was determined using ChIP. ChIP data are shown as differential occupancy fold changes. Data are from one experiment representative of six (a), three (b–d) or two (e–h) independent experiments. Each experiment (d,g,h) was performed in triplicate (n=3). Data are mean+s.d. Figure 3: Linker-phosphorylated Smad2 (S255)–STAT3–p300 complex transactivates the Rorc and Il17a . Interactions of endogenous proteins in T H 17 cells and exogenous proteins in 293T cells were determined by PLA. PLA signals ( a – c , f ) were quantified using the BlobFinder software (scale bars, 10 μm; nucleus, black; cytoplasm, white, n =10 fields). ( a ) Endogenous interaction between Smad2 and STAT3 in T H 17 cells. ( b ) Effects of truncated mutations in Smad2 on the interaction with STAT3 in 293T cells. ( c ) Effects of linker domain variations in Smad2 on the interaction with STAT3 in 293T cells. ( d ) Effects of Smad2 (S255A) on STAT3-induced activation of the Rorc promoter and the Il17a promoter constructs transfected in T H 17 cells were analysed by luciferase assay. ( e ) Flow cytometry analyses of IL-17A + RORγt + CD4 + T cells transduced with the indicated DNA constructs using Nucleofector ( n =2). ( f ) Endogenous interactions between p300 and Smad2 or STAT3 in T H 17 cells were determined using PLA. ( g ) Effects of p300 on Smad2/STAT3-induced activation of the Rorc promoter (white) and the Il17a promoter (black) constructs transfected in 293T cells were analysed by luciferase assay. ( h ) Binding of Smad2 (white) and p300 (black) to the proximal promoter regions of the Rorc gene and the Il17a gene in T H 17 cells was determined using ChIP. ChIP data are shown as differential occupancy fold changes. Data are from one experiment representative of six ( a ), three ( b – d ) or two ( e – h ) independent experiments. Each experiment ( d , g , h ) was performed in triplicate ( n =3). Data are mean+s.d. Full size image The histone acetyl-transferase p300 is a crucial transcription co-activator of Smads [9] , [31] . PLA showed that STAT3 and pSmad2L, but not pSmad2C, had the close proximity with p300 in T H 17 cells ( Fig. 3f ). Luciferase reporter assays confirmed that p300 further enhanced Smad2/STAT3-induced activation of the Rorc and Il17 a promoters in 293T cells ( Fig. 3g ). Smad2, STAT3 and p300 bound to the same sites in the proximal promoters of the Rorc and Il17a genes in T H 17 cells ( Fig. 3h ). Thus, pSmad2L (Ser255) forms complex with p300 and STAT3 to bind to the proximal promoter of the Rorc and Il17a genes. Unphosphorylated Smad3 suppresses T H 17 differentiation We investigated the mechanism how Smad3 functions as a transcription co-repressor of STAT3. PLA confirmed the endogenous close proximity between Smad3 and STAT3 in T H 17 cells ( Fig. 4a ). Unlike R-Smads, Smad4 did not interact with STAT3 ( Fig. 4a ). Although STAT5 and STAT3 oppositely regulate T H 17 differentiation by binding the multiple common sites across the locus encoding IL-17 (ref. 27 ), neither Smad2 nor Smad3 interacted with STAT5 ( Supplementary Fig. 11 ). Furthermore, interactions between Smad2/3 and STAT3 were as significant as the established interaction controls: pSmad2/3C-Smad4 (refs 9 , 10 ) and Smad2/3–RORγt [18] , [21] ( Supplementary Fig. 12 ). PLA and immunoprecipitation of 293T cells transfected with the various deletion mutants of Smad3 showed that Smad3 MH2 deletion mutants (MH1 and MH1+L) [29] failed to bind with STAT3 ( Fig. 4b and Supplementary Fig. 13 ). Thus, the MH2 domain is required for Smad3 to bind STAT3. 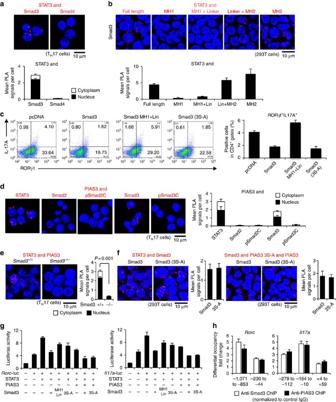Figure 4: C-terminally unphosphorylated Smad3 recruits PIAS3 to act as a transcription co-repressor of STAT3 in TH17 differentiation. Interactions of endogenous proteins in TH17 cells and exogenous proteins in 293T cells were determined using PLA. PLA signals (a,b,d–f) were quantified using the BlobFinder software (scale bars, 10 μm; nucleus, black; cytoplasm, white,n=10 fields). (a) Endogenous interactions between Smad3/Smad4 and STAT3 in TH17 cells. (b) Effects of truncated mutations in Smad3 on the interaction with STAT3 in 293T cells. (c) Flow cytometry analyses of IL-17A+RORγt+CD4+T cells transduced with the indicated DNA constructs using Nucleofector (n=4). (d) Endogenous interactions between PIAS3 and STAT3/Smad2/Smad3 in TH17 cells. (e) Endogenous interaction between PIAS3 and STAT3 inSmad3+/+, −/−TH17 cells. (f) Effects of Smad3 C-terminal mutation on the interaction with STAT3 (left) or the interaction with PIAS3 (right) in 293T cells. (g) Effects of PIAS3, Smad3 MH2 deletion and Smad3 C-terminal mutation on STAT3-induced activation of theRorcpromoter and theIl17apromoter constructs transfected in TH17 cells were determined using the luciferase assay. (h) Binding of Smad3 (white) and PIAS3 (black) to theRorcand theIl17apromoter regions in TH17 cells was determined using ChIP (differential occupancy fold changes). A representative of six (a), three (b,f,g), four (c,d) or two (e,h) independent experiments is shown. Each experiment (g,h) was performed in triplicate (n=3). Data are mean+s.d. or mean+s.d. withPvalues (e, unpaired Student’st-test). Figure 4: C-terminally unphosphorylated Smad3 recruits PIAS3 to act as a transcription co-repressor of STAT3 in T H 17 differentiation. Interactions of endogenous proteins in T H 17 cells and exogenous proteins in 293T cells were determined using PLA. PLA signals ( a , b , d – f ) were quantified using the BlobFinder software (scale bars, 10 μm; nucleus, black; cytoplasm, white, n =10 fields). ( a ) Endogenous interactions between Smad3/Smad4 and STAT3 in T H 17 cells. ( b ) Effects of truncated mutations in Smad3 on the interaction with STAT3 in 293T cells. ( c ) Flow cytometry analyses of IL-17A + RORγt + CD4 + T cells transduced with the indicated DNA constructs using Nucleofector ( n =4). ( d ) Endogenous interactions between PIAS3 and STAT3/Smad2/Smad3 in T H 17 cells. ( e ) Endogenous interaction between PIAS3 and STAT3 in Smad3 +/+, −/− T H 17 cells. ( f ) Effects of Smad3 C-terminal mutation on the interaction with STAT3 (left) or the interaction with PIAS3 (right) in 293T cells. ( g ) Effects of PIAS3, Smad3 MH2 deletion and Smad3 C-terminal mutation on STAT3-induced activation of the Rorc promoter and the Il17a promoter constructs transfected in T H 17 cells were determined using the luciferase assay. ( h ) Binding of Smad3 (white) and PIAS3 (black) to the Rorc and the Il17a promoter regions in T H 17 cells was determined using ChIP (differential occupancy fold changes). A representative of six ( a ), three ( b , f , g ), four ( c , d ) or two ( e , h ) independent experiments is shown. Each experiment ( g , h ) was performed in triplicate ( n =3). Data are mean+s.d. or mean+s.d. with P values ( e , unpaired Student’s t -test). Full size image PIAS3 belongs to the mammalian protein inhibitor of activated STAT (PIAS) protein family, which represses STAT3-dependent transcriptional activation by blocking the DNA-binding activity of STAT3, regardless of its small ubiquitin-like modifier-E3 ligase activity [32] . Overexpression of Smad3, the deletion mutant lacking MH2 domain or the C-terminal mutant in T H 17 cells show that the Smad3 MH2 domain, but not the C-terminal SSXS motif, is functionally responsible for the suppression of T H 17 differentiation ( Fig. 4c ). Because PIAS3 interacts with Smad3 at its C-terminal domain [33] , we examined whether Smad3 recruits PIAS3 to repress STAT3-induced transcription of the Rorc and Il17a genes. PIAS3 showed the close proximity with both STAT3 and Smad3, but not with C-terminally phosphorylated Smad3 (pSmad3C) or Smad2 in T H 17 cells ( Fig. 4d ). STAT3–PIAS3 interaction was completely abolished in Smad3 −/− T H 17 cells ( Fig. 4e ). A mutant of serine residues to alanine in the Smad3 SSXS motif, Smad3 (3S-A), was yet capable of binding with STAT3 and PIAS3 in 293T cells ( Fig. 4f ). Consistently, when co-transfected with PIAS3 in T H 17 cells, Smad3 (3S-A) was able to suppress STAT3-induced activation of the Rorc and Il17a reporters ( Fig. 4g ). ChIP revealed that PIAS3 and Smad3, but not pSmad3C, bound to the same sites in the Rorc and Il17a promoters ( Fig. 4h and Supplementary Fig. 14 ). Thus, C-terminal phosphorylation is not required for Smad3 to bind with STAT3 and PIAS3. Overexpression of PIAS3 suppressed T H 17 differentiation, whereas knockdown of PIAS3 by siRNA abolished the binding of Smad3 to the Rorc and Il17a promoter regions, although T H 17 differentiation was unaltered by knockdown of PIAS3 presumably because relatively predominant binding of Smad2 over Smad3 in the absence of PIAS3 transactivated the Rorc and Il17a genes ( Supplementary Fig. 15 ). These data indicate that unphosphorylated Smad3C in cooperation with PIAS3 represses STAT3-induced transcription of the Rorc and Il17a genes. ERK phosphorylates Smad2 linker in T H 17 differentiation Previous studies have paid attention to C-terminal phosphorylation of R-Smads as TGF-β signalling mediators in T H 17 differentiation [18] , [19] , [20] , [21] , [22] , [23] . However, pSmad2L (Ser255) and unphosphorylated Smad3 are not involved in the canonical C-terminally phosphorylated R-Smad/Smad4-mediated TGF-β signalling. Three clustered serine residues in the linker regions of Smad2 (Ser245/250/255) are the phosphorylation sites for MAPKs (ERK, JNK and p38) [10] , [11] , [12] , [13] , [34] . Because MAPKs are shared by TGF-β, IL-6 and TCR, we sought to identify the MAPK responsible for Smad2 linker phosphorylation in T H 17 differentiation. Signal intensities of TGF-β, IL-6 and TCR have been reported to correlate with the extent of T H 17 differentiation [3] , [4] , [16] . Therefore, we treated CD4 + T cells under T H 17-polarizing condition with various concentrations of TGF-β, IL-6 and anti-CD3 antibody. We confirmed that higher doses of TGF-β1, anti-CD3 antibody and IL-6 induced more T H 17 differentiation ( Fig. 5a and Supplementary Figs 16a and 17a ). Percentages of IL-17A + RORγt + CD4 + T cells were directly proportional to phosphorylation of Smad2L ( Fig. 5b and Supplementary Figs 16b and 17b ) and ERK, but not to the phosphorylation of JNK or p38 ( Fig. 5c and Supplementary Figs 18 and 19 ). 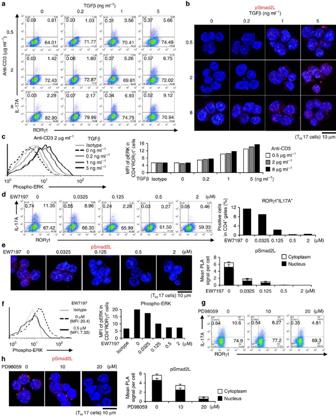Figure 5: ERK induces Smad2 linker phosphorylation that facilitates TH17 differentiation. Purified CD4+T cells were activated under TH17-polarizing condition with the indicated doses of TGF-β1 and plate-coated anti-CD3 antibody, or small molecule inhibitors (EW-7197, ALK5 inhibitor; PD98059, MEK inhibitor) for 3 days. (a) Flow cytometry analyses of IL-17A+RORγt+CD4+T cells treated with TGF-β1 and plate-coated anti-CD3 antibody. (b) Endogenous expression of pSmad2L in TH17 cells treated with TGF-β1 and plate-coated anti-CD3 antibody was determined using PLA. (c) Flow cytometry analyses of phospho-ERK in TH17 cells treated with TGF-β1 and plate-coated anti-CD3 antibody. (d) Flow cytometry analyses of IL-17A+RORγt+CD4+T cells treated with EW-7197. (e) Endogenous expression of pSmad2L in TH17 cells treated with EW-7197 was determined using PLA. (f) Flow cytometry analyses of phospho-ERK in TH17 cells treated with EW-7197. (g) Flow cytometry analyses of IL-17A+RORγt+CD4+T cells treated with PD98059. (h) Endogenous expression of pSmad2L in TH17 cells treated with PD98059 was determined using PLA. The values of the mean fluorescence intensity (MFI) are shown in graphs. PLA signals (b,e,h) were quantified using the BlobFinder software (scale bars, 10 μm; nucleus, black; cytoplasm, white,n=10 fields). Data are representative of two (a–h) independent experiments. Data are mean+s.d. Figure 5: ERK induces Smad2 linker phosphorylation that facilitates T H 17 differentiation. Purified CD4 + T cells were activated under T H 17-polarizing condition with the indicated doses of TGF-β1 and plate-coated anti-CD3 antibody, or small molecule inhibitors (EW-7197, ALK5 inhibitor; PD98059, MEK inhibitor) for 3 days. ( a ) Flow cytometry analyses of IL-17A + RORγt + CD4 + T cells treated with TGF-β1 and plate-coated anti-CD3 antibody. ( b ) Endogenous expression of pSmad2L in T H 17 cells treated with TGF-β1 and plate-coated anti-CD3 antibody was determined using PLA. ( c ) Flow cytometry analyses of phospho-ERK in T H 17 cells treated with TGF-β1 and plate-coated anti-CD3 antibody. ( d ) Flow cytometry analyses of IL-17A + RORγt + CD4 + T cells treated with EW-7197. ( e ) Endogenous expression of pSmad2L in T H 17 cells treated with EW-7197 was determined using PLA. ( f ) Flow cytometry analyses of phospho-ERK in T H 17 cells treated with EW-7197. ( g ) Flow cytometry analyses of IL-17A + RORγt + CD4 + T cells treated with PD98059. ( h ) Endogenous expression of pSmad2L in T H 17 cells treated with PD98059 was determined using PLA. The values of the mean fluorescence intensity (MFI) are shown in graphs. PLA signals ( b , e , h ) were quantified using the BlobFinder software (scale bars, 10 μm; nucleus, black; cytoplasm, white, n =10 fields). Data are representative of two ( a – h ) independent experiments. Data are mean+s.d. Full size image To confirm whether TβRI-mediated phosphorylation of Smad2L is required for T H 17 differentiation, we treated CD4 + T cells under T H 17-polarizing condition with specific inhibitors against TβRI [35] at the doses that maintain cell viability ( Supplementary Fig. 20 ). A potent selective ATP-competitive inhibitor of TβRI kinase (activin receptor-like kinase5: ALK5), EW-7197 (refs 35 , 36 ) completely suppressed T H 17 differentiation at the dose of 0.5 μM ( Fig. 5d ). Treatment with EW-7197 suppressed pSmad2L ( Fig. 5e ) and phosphorylation of ERK, but not phosphorylation of JNK and p38 ( Fig. 5f and Supplementary Fig. 21 ). One of the prototype ALK5 inhibitors, SB-505124, inhibits TGF-β-induced activation of MAPKs without altering ALK5-independent MAP kinase pathways [37] . A more highly selective ALK5 inhibitor, EW-7197, does not directly inhibit MEK1 and ERK1 (ref. 35 ). Therefore, inhibitory effect of EW-7197 on ERK phosphorylation is ALK5-specific. Culture media containing IL-6, IL-23 and IL-1β is sufficient to induce T H 17 in the absence of TGF-β (ref. 38 ). However, EW-7197 inhibited, whereas TGF-β1 enhanced T H 17 differentiation along with ERK phosphorylation even under this culture condition ( Supplementary Fig. 22 ). These results suggest that TGF-β-TβRI signal phosphorylates ERK and Smad2L in T H 17 cells. To confirm whether ERK-mediated phosphorylation of Smad2L is required for T H 17 differentiation, we next treated CD4 + T cells under T H 17-polarizing condition with specific inhibitors against MAPKs at the doses that maintain cell viability ( Supplementary Figs 23 and 24 ). A MEK inhibitor PD98059 suppressed T H 17 differentiation in a dose-dependent manner ( Fig. 5g and Supplementary Fig. 23 ), whereas a JNK inhibitor SP600125 or p38 inhibitor SB203580 did not affect T H 17 differentiation ( Supplementary Fig. 24 ). PD98059 showed the similar effects with EW-7197 on pSmad2L ( Fig. 5h ). Specific inhibition of MAP kinase by the corresponding inhibitor was confirmed ( Supplementary Fig. 25 ). Taken together, ERK-mediated Smad2 linker phosphorylation is responsible for T H 17 differentiation and the concentrations of TGF-β, TCR and IL-6 determine the intensities of Smad2 linker phosphorylation and the extent of T H 17 differentiation. R-Smad–STAT3 interactions balance T H 17 differentiation We next examined the effects of intensities and inhibitions of TGF-β/IL-6/TCR signals on the interactions of STAT3 with pSmad2L or unphosphorylated Smad3C in T H 17 cells. Higher doses of TGF-β1, IL-6 and anti-CD3 antibody significantly upregulated pSmad2L–STAT3 interactions with little changes in Smad3–STAT3 interactions ( Fig. 6a,b and Supplementary Fig. 26 ). By contrast, treatments with EW-7197 or PD98059 significantly downregulated pSmad2L–STAT3 interactions ( Fig. 6c,e ), whereas upregulated Smad3–STAT3 interactions ( Fig. 6d,f ). Interactions of pSmad2L and STAT3 were directly proportional, whereas interactions of unphosphorylated Smad3C and STAT3 were inversely proportional to T H 17 differentiation of EW-7197- or PD98059-treated CD4 + T cells ( Figs 5d,g and 6c–f ). These data suggest that the balances between STAT3-interacting pSmad2L and STAT3-interacting unphosphorylated Smad3C determine the extent of T H 17 differentiation. 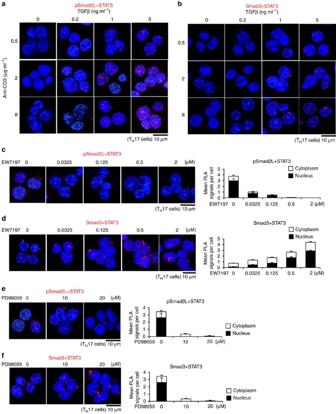Figure 6: R-Smad–STAT3 interaction balances correlate with TH17 differentiation. Purified CD4+T cells were activated under TH17-polarizing condition with the indicated doses of TGF-β1 and plate-coated anti-CD3 antibody, or small molecule inhibitors (EW-7197, ALK5 inhibitor; PD98059, MEK inhibitor) for 3 days. Interactions of endogenous proteins in TH17 cells were determined with PLA. PLA signals (a–f) were quantified using the BlobFinder software (scale bars, 10 μm; nucleus, black; cytoplasm, white,n=10 fields). (a) pSmad2L and STAT3, (b) Smad3 and STAT3 in TH17 cells treated with the indicated doses of TGF-β1 and plate-coated anti-CD3 antibody. (c) pSmad2L and STAT3, (d) Smad3 and STAT3 in TH17 cells treated with the indicated doses of EW-7197. (e) pSmad2L and STAT3, (f) Smad3 and STAT3 in TH17 cells treated with the indicated doses of PD98059. Data are representative of two independent experiments. Data are mean+s.d. Figure 6: R-Smad–STAT3 interaction balances correlate with T H 17 differentiation. Purified CD4 + T cells were activated under T H 17-polarizing condition with the indicated doses of TGF-β1 and plate-coated anti-CD3 antibody, or small molecule inhibitors (EW-7197, ALK5 inhibitor; PD98059, MEK inhibitor) for 3 days. Interactions of endogenous proteins in T H 17 cells were determined with PLA. PLA signals ( a – f ) were quantified using the BlobFinder software (scale bars, 10 μm; nucleus, black; cytoplasm, white, n =10 fields). ( a ) pSmad2L and STAT3, ( b ) Smad3 and STAT3 in T H 17 cells treated with the indicated doses of TGF-β1 and plate-coated anti-CD3 antibody. ( c ) pSmad2L and STAT3, ( d ) Smad3 and STAT3 in T H 17 cells treated with the indicated doses of EW-7197. ( e ) pSmad2L and STAT3, ( f ) Smad3 and STAT3 in T H 17 cells treated with the indicated doses of PD98059. Data are representative of two independent experiments. Data are mean+s.d. Full size image In summary, the TGF-β/IL-6/TCR–pERK–pSmad2L (Ser255) axis is the positive regulator, whereas unphosphorylated Smad3C–PIAS3 complex is the negative regulator of STAT3-induced transcriptional processes for T H 17 differentiation ( Fig. 7 ). 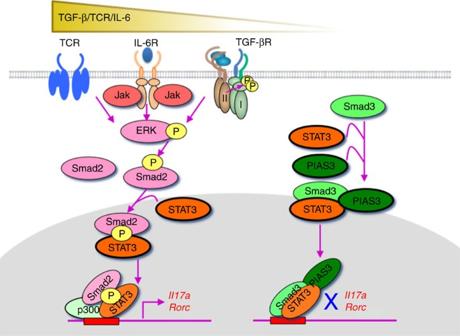Figure 7: TGF-β R-Smads, Smad2 and Smad3, oppositely regulate TH17 differentiation as transcription cofactors of STAT3. ERK-phosphorylated Smad2L (S255)/STAT3/p300 activates, whereas unphosphorylated Smad3C/STAT3/PIAS3 represses the transcription of theRorcandIl17agenes. Figure 7: TGF-β R-Smads, Smad2 and Smad3, oppositely regulate T H 17 differentiation as transcription cofactors of STAT3. ERK-phosphorylated Smad2L (S255)/STAT3/p300 activates, whereas unphosphorylated Smad3C/STAT3/PIAS3 represses the transcription of the Rorc and Il17a genes. Full size image We discovered that Smad2 and Smad3 oppositely regulated STAT3-induced T H 17 differentiation through the novel direct signalling networks. Transmodulation between the SMAD and STAT signalling pathways balances the interplay between TGF-β and various cytokines. Indirect crosstalk between SMAD and STAT was first reported as the inhibition of Smad3/4-mediated TGF-β signalling by Jak1-STAT1-mediated interferon (IFN)-γ signalling via induction of the inhibitory Smad, Smad7, which prevents TβRI-induced C-terminal phosphorylation of Smad3 (ref. 39 ). Direct crosstalk between SMAD and STAT was discovered as the synergistic signalling of leukaemia inhibitory factor and bone morphogenic protein-2, one of the TGF-β superfamily cytokines, via the STAT3–Smad1 complex bridged by p300 in fetal neural cells [40] . Direct crosstalk between Smad3 and STAT3 was reported as the augmentation of IL-6-STAT3-mediated transactivation by TGF-β via interaction of the STAT3–pSmad3C complex bridged by p300 in hepatoma cells [41] . This study clarified the mechanisms whereby R-Smads–STAT3 networks modulate T H 17 differentiation; pSmad2L (Ser255) serves as STAT3 co-activator in combination with p300, a co-activator of various transcription factors including both Smads and STAT3 (refs 27 , 31 ), whereas unphosphorylated Smad3C serves as the STAT3 co-repressor in combination with PIAS3, a negative regulator of STAT3-induced transcription [32] . The preceding reports and our findings indicate that SMAD–STAT signalling networks are highly cell-type-specific and context-dependent. Because of the relatively low DNA-binding affinity of Smad3 and lack of DNA-binding ability of Smad2, they interact with a wide variety of DNA-binding proteins to co-regulate the target genes. Recently, genome-wide transcriptome analyses have elucidated the diverse regulatory networks of Smad2/3 with cell-type-specific master transcription factors and/or DNA-binding cofactors in variety of cells [42] . The thorough iterative approach to delineate the T H 17 global transcriptional regulatory network shows that STAT3 works as one of the key activators of the initial transcriptional programme, RORγt works as an expression modulator and Smad3 is the negative regulators [43] . It is noteworthy that a histone demethylase, JMJD3 (KDM6B) regulates the expression of numerous targets of RORγt and STAT3 (ref. 43 ) because JMJD3 causes a loss of the H3K27me3-repressive epigenetic mark by interacting with R-Smads at their target sites [42] . Therefore, it is possible that Smad2 may interact with JMJD3 to induce active chromatin state for T H 17 regulation in the same manner with Nodal-Smad2/3 signalling in embryonic development [44] ( Supplementary Fig. 8 ). Further studies are required to elucidate the details of divergent context-dependent SMAD–STAT signalling networks implicated by genome-wide transcriptome analyses. We further uncovered the novel roles of R-Smads with noncanonical phosphorylation status in networking with STAT3: linker phosphorylated Smad2 as a STAT3 co-activator and unphosphorylated Smad3 as a STAT3 co-repressor. Serine/threonine-rich R-Smad linker regions contain multiple phosphorylation sites by proline-directed protein kinases such as MAPKs, glycogen synthase kinase 3 and cyclin-dependent kinase family [11] , [12] , [13] . Linker residues Ser245/250/255, Thr220 in Smad2 and Ser204/208/213, Thr179 in Smad3 are the sites for phosphorylation [12] , [13] . Three clustered serine residues are preferred phosphorylation sites for ERK, JNK and p38 in response to receptor tyrosine kinases and proinflammatory cytokines, whereas threonine residues are preferred phosphorylation sites for cyclin-dependent kinase family in response to TGF-β. TβRI possesses the intrinsic tyrosine kinase activity to directly induce activation of MAPK pathways and subsequent phosphorylation of R-Smad linker residues in addition to the serine/threonine kinase activity to phosphorylate R-Smads in their conserved C-terminal SSXS motif [5] , [11] . Mitogens and hyperactive Ras induce ERK-mediated linker phosphorylation of Smad2 at Ser245/250/255/Thr220 and Smad3 at Ser204/208/Thr179 (refs 12 , 13 ). Therefore, roles of R-Smad linker phosphorylation in carcinogenesis have been investigated intensively [11] , [12] , [13] . Central role of ERK in TCR signals [15] , [24] suggests the important roles of R-Smad linker phosphorylation in T-cell signalling network. Thus far, MEKK2/3-ERK1/2 signalling has been reported to induce pSmad3L, which negatively regulates canonical TGF-β signalling for T H 17 differentiation [45] . Because we found that Smad3 linker region was not involved in STAT3-induced T H 17 differentiation ( Fig. 4b ), the mechanisms how pSmad3L regulates T H 17 differentiation are independent of STAT3. By contrast to phosphorylated Smads, very little has been known about physiological functions of unphosphorylated R-Smads. It has been reported that PIAS3 enhances TGF-β-induced transcriptional activity of C-terminally phosphorylated Smad3 by recruiting p300 and CBP in COS and 293T cells [33] . By contrast, we discovered that unphosphorylated Smad3C due to less TGF-β signalling was required for PIAS3 to function as a co-repressor of STAT3 (ref. 32 ). Recent genome-wide studies implicate that unphosphorylated Smad3 may bind to some cell-type-specific transcription factors in both TGF-β-dependent and TGF-β-independent manners [42] , [46] , [47] . Our finding shed light on as-yet-unrecognized functions of unphosphorylated Smad3 as a transcription cofactor. The discovery of a new proinflammatory effector T-cell subset, T H 17, revised the functions of TGF-β, which had been long considered as the most potent immunosuppressive cytokine. TGF-β has been identified as the requisite factor for T H 17 differentiation in combination with IL-6 and other proinflammatory cytokines such as IL-21, IL-23, IL-1β and tumour-necrosis factor-α (TNF-α) [3] , [4] , [6] . However, as functions of TGF-β have been frequently described as dual, bidirectional, pleiotropic, complex or contextual [5] , [9] , [10] , [11] , [12] , [13] , the roles of TGF-β in T H 17 differentiation have become controversial [18] , [19] , [20] , [21] , [22] , [23] . Requirement of TGF-β for T H 17 differentiation remains contradictory, indispensable [4] or dispensable [38] . Our results provide explanation for these conflicting reports. TGF-β ligand-independent T H 17 differentiation is possible because Smad2 linker phosphorylation could be induced by ERK signals downstream of the IL-6 receptor and TCR. However, significantly more effective inhibitory effect of the ALK5 inhibitor than that of a MEK inhibitor suggests that the TβRI–pERK–pSmad2L axis is more efficient than the non-TGF-β growth-stimulatory signal-pERK-pSmad2L axis for T H 17 differentiation. Nonetheless, the report showing the dispensability of TGF-β demonstrates that TGF-β induces significantly more T H 17 differentiation [38] . Likewise, our results provide explanations for the discrepancies in the reported roles of Smads in T H 17 differentiation [18] , [19] , [20] , [21] , [22] , [23] . Our data are consistent with the previous reports showing that Smad2 is a positive regulator and Smad3 is a negative regulator of T H 17 differentiation, although the mechanisms of actions are distinct [18] , [19] , [20] , [21] . It has been reported that TGF-β signalling via Smad2 indirectly induced STAT3 phosphorylation by inducing the expression of mRNA and protein of IL-6Rα (ref. 19 ); however, we could not confirm the differences in IL-6Rα mRNA expression in our systems ( Supplementary Fig. 7 ). It has been reported that Smad3 interacted with RORγt and decreased its transcriptional activity [21] . We confirmed that not only Smad3 but also Smad2 interacted with RORγt ( Supplementary Fig. 12 ). Whether RORγt forms the complex with STAT3 and R-Smads remains to be determined. Our data also suggest that the signalling intensity balances of TCR, co-stimulation, IL-6, TGF-β and other cytokines could yield the seeming dispensability of R-Smads [22] , [23] because of their opposing effects. The signalling balances between TβRI-PKCα-mediated C-terminal phosphorylation of R-Smads [48] and pERK-pSmad2L may be also crucial for T H 17 differentiation. An ALK5 inhibitor is efficacious against a mouse type II collagen antibody-induced arthritis model [49] . Our results of a CIA model showed the promoting role of pSmad2L at Ser255 and the suppressive role of unphosphorylated Smad3 in the arthritogenic T H 17 differentiation. Therefore, inhibiting phosphorylation of Smad2 linker or Smad3 C-terminus may have therapeutic utility for RA and various T H 17-related inflammatory diseases. Considering the crucial roles of SMADs and STATs in cell regulation, homeostasis and the pathogenesis of various diseases such as infection, cancers, fibrosis and inflammation, our findings will lead to the elucidation of cytokine signalling networks in various settings. In summary, we show the novel signalling networks of R-Smads and STAT3 for T H 17 differentiation, which revise the classical linear signalling cascades [50] . Mice Smad2 3loxp/3loxp mice targeting exons 9 and 10 (ref. 51 ), Smad3 ex8/ex8 mice targeting exon 8 (ref. 52 ) were generated as described on Sv129 × C57BL/6J background and backcrossed to C57BL/6J mice (Nihon SLC) for eight generations. For in vitro experiments, Smad3 ex8/ex8 mice were backcrossed to C57BL/6J background for four generations. We used Smad3 +/− mice because Smad3 −/− mice develop osteoarthritis, bone malformation [53] and impaired mucosal immunity [52] , and the embryonic lethality of Smad3 −/− mice in the C57BL/6 background was extremely high ( Supplementary Fig. 27 ), similarly with Tgf-β1 −/− mice [54] . Cd4Cre transgenic mice [55] were purchased from Jackson Laboratories. Mx-1Cre transgenic mice [56] were kindly provided by Dr Masayuki Yamamoto (Tohoku University, Japan). For Mx-1Cre mice at 2–3 weeks of age, gene deletion was induced by intraperitoneal injections of 250 μg polyI:C dissolved in sterile saline at 2-day intervals for a total of three injections [56] . For immunophenotyping, spleens and superficial lymph nodes (cervical, axillary, brachial and inguinal) from the female mice aged between 12 and 16 weeks of age were used (age- and sex-matched, no randomized). All animals were maintained and used for experiments according to the ethical guidelines for animal experiments and the safety guidelines for gene manipulation experiments at the Konkuk University, Republic of Korea, University of Tsukuba, Japan, Tokyo Medical University, Japan under approved animal study protocols. CIA For induction of CIA, we used the immunization protocol for C57BL/6 strain (H-2b) [57] . Briefly, mice aged between 8 and 10 weeks of age were injected intradermally at several sites into the base of the tail and back with type II collagen (Sigma-Aldrich, Cat. no. C9301) emulsified in complete Freund adjuvant: incomplete Freund adjuvant (GIBCO), heat-killed mycobacterium tuberculosis (Difco Laboratories) on day −21 and the same injection was repeated on day 0 ( Fig. 1a and Supplementary Fig. 2 ). Arthritis development in each paw was scored by macroscopic evaluation [58] as follows: (0) no change, (1) erythema and mild swelling confined to the ankle, (2) erythema and mild swelling from the ankle to midfoot, (3) moderate swelling and (4) severe swelling. The maximum score per mouse is 16. The investigators (M.M., K.S., S.N. and J.S.H.) were blinded to the genotypes. Ten to twenty mice/genotype were used ( Fig. 1 legend and Supplementary Fig. 2 legend). Mice were dissected 2 weeks after the second immunization to evaluate the draining lymph nodes (popliteal, inguinal, axillary and brachial). Histological analysis Paws from collagen-immunized mice were harvested, fixed in 10% neutral-buffered formalin, decalcified, dehydrated with 70% ethanol, embedded in paraffin and sectioned at 3 μm. Sections were stained with haematoxylin and eosin, toluidine blue or safranin O. For immunohistochemistry, sections were stained with rat anti-CD4 (Abcam, Cat. no. ab25475, 1:50), rabbit anti-RORγt (Abcam, Cat. no. ab78007, 1:50) and rabbit anti-IL-17A (Abcam, Cat. no. ab79056, 1:50) antibodies. Slides were observed using an optical microscope, DM5000B (Leica). Flow cytometry analyses Fluorophore-conjugated antibodies were purchased from BD Pharmingen and eBioscience. CD16/32 were blocked by Fc-Block (BD Pharmingen, Cat. no. 553142) and isotype-matched control antibodies were used in each experiment. For cytokine intracellular staining, cultured cells or freshly isolated cells from CIA mice were treated with 5 ng ml −1 of phorbol-12-myristate 13-acetate (Sigma-Aldrich) and 500 ng ml −1 of ionomycin (Sigma-Aldrich) in the presence of GolgiPlug (BD Pharmingen) for the last 4 h of culture. For intracellular staining, cultured cells were fixed with the Cytoperm/Cytofix kit (BD Pharmingen). For Foxp3 staining, the Foxp3 staining kit (eBioscience, Cat. no. 00-5523-00) was used. Stained cells were acquired and analysed using LSR II (BD) and FlowJo software (Tree Star Inc.). T-cell stimulation in vitro CD4 + T cells from superficial lymph nodes and spleens were enriched using T-cell enrichment columns (R&D Systems) and MACS system (Miltenyi Biotech). Purity was confirmed as >90% using LSR II. In some experiments, CD44 low CD62L high CD4 + T cells were sorted with FACSAria (BD) and the purity was >98%. Purified CD4 + T cells were stimulated by plate-coated anti-CD3 (2.0 μg ml −1 ; BD Pharmingen, Cat. no. 553057) and soluble anti-CD28 antibodies (5.0 μg ml −1 ; BD Pharmingen, Cat. no. 553294) with mIL-6 (50 ng ml −1 ), TGF-β1 (1 ng ml −1 ; Peprotech), anti-mouse IL-4 (10 μg ml −1 ; Biolegend, Cat. no. 504108) and anti-mouse IFN-γ antibodies (10 μg ml −1 ; BioLegend, Cat. no. 505812) in 10% FCS RPMI 1640 media supplemented with penicillin and streptomycin (HyClone) for T H 17 differentiation for 3–4 days [3] . In some experiments, Purified CD4 + T cells were stimulated by the indicated doses of plate-coated anti-CD3, TGF-β1 and mIL-6, or by plate-coated anti-CD3 (10.0 μg ml −1 ; BD Pharmingen, Cat. no. 553057), soluble anti-CD28 antibodies (5.0 μg ml −1 ; BD Pharmingen, Cat. no. 553294), IL-1β (10 ng ml −1 ; Peprotech), IL-23 (10 ng ml −1 ; Peprotech) and the neutralizing antibodies described above, or by the indicated doses of various small molecule inhibitors: EW-7197 (ALK5 inhibitor) from Dr Dae-Kee Kim, PD98059 (MEK inhibitor), SP600125 (JNK inhibitor) and SB203580 (p38 inhibitor; Sigma-Aldrich). STAT3 siRNA (Dharmacon), PIAS3 siRNA (Santa Cruz), DNA constructs: Smad2, Smad2 (S255A), Smad3, Smad3 (3S-A) and Smad3 (MH1+L) from Dr Koichi Matsuzaki and Dr Takeshi Imamura, PIAS3 (Addgene, submitted by Shuai) and pcDNA or control RNA were transfected to purified CD4 + T cells using the 4D-Nucleofector and Amaxa Mouse T-cell Nucleofector kit (Lonza) before the cell culture. RNA isolation and quantitation of mRNA using real-time RT–PCR Total RNA was extracted using Trizol according to the manufacturer’s instructions (Invitrogen). RNA was reverse-transcribed with the cDNA reverse transcription kit (Invitrogen). Amount of cDNA was quantitated with SYBR green (Applied Biosystems) real-time PCR using ABI 7900 and ABI 7300 machines (Applied Biosystems). The primers are described in Supplementary Table 1 . Western blot analysis and immunoprecipitation 293T cells (ATCC-CRL-3216) were transfected using PEI with STAT3 (Addgene, submitted by J. Darnell), FLAG-tagged Smad2 (full length, MH1, MH1+Linker, MH2+Linker, MH2, Y220V, S245A, S250A, S255A) and FLAG-tagged Smad3 (full length, MH1, MH1+Linker, MH2+Linker, MH2, 3S-A) from Dr Koichi Matsuzaki and Dr Takeshi Imamura. Cells were lysed with lysis buffer (PBS containing 0.5% Triton X-100, 20 mM HEPES (pH 7.4), 150 mM NaCl, 12.5 mM β-glycerol phosphate, 1.5 mM MgCl2, 10 mM NaF, 2 mM dithiothreitol, 1 mM NaOV, 2 mM EGTA, 1 mM phenylmethylsulphonyl fluoride (PMSF) and protease inhibitor cocktail) were electrophoresed on 10% SDS–polyacrylamide gel and transferred to the polyvinylidene difluoride (PVDF) membrane, and probed with antibodies against phospho-Smad2 (Abcam, Cat. no. ab53100, 1:1,000 dilution), phospho-Smad3 (Abcam, Cat. no. ab51451, 1:1,000 dilution), Smad2 (Santa Cruz, Cat. no. sc-101153, 1:1,000 dilution), Smad3 (Santa Cruz, Cat. no. sc-101154, 1:1,000 dilution), Smad4 (Santa Cruz, Cat. no. sc-7966, 1:1,000 dilution) and β-actin (Santa Cruz, Cat. no. sc-7210, 1:10,000 dilution). Blots were visualized using an electrochemiluminescence kit (GE Healthcare). For immunoprecipitation, the lysates were cleared using centrifugation at 16,000 g for 10 min, incubated with protein A/G agarose beads and with anti-STAT3 antibody (Santa Cruz, Cat. no. sc-7179, 2.0 μg per 1 ml of cell lysate) at 4 °C for 12–16 h. The beads were washed three times with lysis buffer and immunoprecipitates were separated from the beads by adding 2 × sample buffer and boiled. SDS–PAGE-separated immunoprecipitates were transferred on PVDF membranes. The membranes were denatured with denaturation buffer containing 6 M guanidine chloride, 20 mM Tris (pH 7.5), 100 mM PMSF and 5 mM β-mercaptoethanol at 4 °C for 30 min and washed three times with TBST. The membranes were blocked with 5% BSA and incubated with anti-FLAG antibody (Biomol, Cat. no. ADI-SAB-410-0100, 1:1,000 dilution). 293T cells (ATCC-CRL-3216) were confirmed to be mycoplasma-negative using the e-Myco plus Mycoplasma PCR Detection Kit (iNtRON Biotechnology, Cat. no. 25237). PLA CD4 + T cells cultured in T H 17 condition for 3–5 days or 293T cells (ATCC-CRL-3216) transfected with various constructs were fixed on the slides by 3.7% formaldehyde in PBS. The slides were washed, permeabilized by 0.1% Triton X-100 in TBS and blocked by 0.5% BSA. PLA was performed using the Duolink II Fluorescence kit (OLINK) using the rabbit antibodies (1:50 dilution) against: STAT3 (Cell Signaling Technology, Cat. no. 12640), phospho-STAT3 Y705 (Cell Signaling Technology, Cat. no. 9145), phospho-STAT3 S727 (Cell Signaling Technology, Cat. no. 9134), Smad2 (Cell Signaling Technology, Cat. no. 5339), phospho-Smad2C S465/467 (Cell Signaling Technology, Cat. no. 3101), phospho-Smad2L S245/250/255 (Cell Signaling Technology, Cat. no. 3104), Smad3 (Cell Signaling Technology, Cat. no. 9523), phospho-Smad3C S423/425 (Cell Signaling Technology, Cat. no. 9520), RORγt (Abcam, Cat. no. ab78007), PIAS3 (Santa Cruz, Cat. no. sc-14017), Flag (Biomol, Cat. no. ADI-SAB-410-0100) and phospho-Smad3L S208/213 (IBL, Cat. no. JP28029), mouse antibodies (1:50 dilution) against: Smad2/3 (Santa Cruz, Cat. no. sc-133098), Smad4 (Santa Cruz, Cat. no. sc-7966), STAT3 (Santa Cruz, Cat. no. sc-8019) and p300 (Santa Cruz, Cat. no. sc-48343). Target-specific rabbit primary antibodies and the secondary antibodies conjugated with oligonucleotides: PLA probe anti-rabbit PLUS (Sigma-Aldrich, Cat. no. DUO92002) and PLA probe anti-rabbit MINUS (Sigma-Aldrich, Cat. no. DUO92005) or PLA probe anti-mouse PLUS (Sigma-Aldrich, Cat. no. DUO92001) and PLA probe anti-mouse MINUS (Sigma-Aldrich, Cat. no. DUO92004) were used for single recognitions. Two primary antibodies raised in different species and the secondary antibodies conjugated with oligonucleotides: PLA probe anti-rabbit PLUS and PLA probe anti-mouse MINUS were used for double recognitions. After incubation of the slides with Blocking Solution for 30 min at 37 °C, they were incubated with primary antibodies diluted in the Antibody Diluent overnight at 4 °C, in PLA probe solution for 1 h at 37 °C and in Ligation-Ligase solution for 30 min at 37 °C with washing with Wash Buffer A in the interim of each step. The slides were incubated in Amplification-Polymerase solution for 100 min at 37 °C and then washed in Wash Buffer B. The nucleus was stained with DAPI. Then, the slides were dried at room temperature in the dark. Slides were observed using a confocal microscope, LSM700 (Carl Zeiss). PLA signals were quantified using the BlobFinder software (Centre for Image Analysis, Uppsala University). Luciferase assay The 2,000-bp promoter region of RORγt was generated using PCR from genomic C57BL/6 DNA using primers described in Supplementary Table 2 . Products were verified by sequencing and were subcloned into pGL4 firefly luciferase construct (Promega) using NheI, EcoRV sites and XhoI, HindIII sites, respectively. The pGL4 mIL-17 2-kb promoter construct was from Addgene (submitted by W. Strober). The promoter constructs in various combinations with Flag-tagged STAT3 (Addgene, submitted by J. Darnell), Flag-tagged Smads, Flag-tagged Smad mutants, haemagglutinin-tagged p300, Flag-tagged PIAS3 (Addgene, submitted by Shuai) or empty pcDNA3 plasmid were co-transfected with control TK-pRL Renilla plasmid using PEI for 293T cells or using the 4D-Nucleofector and Amaxa Mouse T-cell Nucleofector kit (Lonza) for T H 17 cells. Six hours after transfection, 293T cells (ATCC-CRL-3216) were lysed for the measurement using luminometer. CD4 + T cells were transfected before the cell culture under T H 17-polarizing condition for 4 days. ChIP Chromatin was prepared from 1 × 10 7 CD4 + T cells isolated from C57BL/6 mice, Cd4Cre;Smad2 fl/fl mice, Smad3 −/− mice and the littermate control mice under T H 17-polarizing condition for 3–4 days. Immunoprecipitation was performed with antibodies (1:50 dilution) against Smad2 (Cell Signaling Technology, Cat. no. 5339), Smad3 (Cell Signaling Technology, Cat. no. 9523), phospho-Smad3C S423/425 (Cell Signaling Technology, Cat. no. 9520), Smad4 (Santa Cruz, Cat. no. sc-7966), STAT3 (Santa Cruz, Cat. no. sc-7179), tri-methyl histone H3 Lys4 (Cell Signaling Technology, Cat. no. 9751), tri-methyl histone H3 Lys27 (Cell Signaling Technology, Cat. no. 9733), acetyl histone H3 Lys23 (Millipore, Cat. no. 17–10112) and PIAS3 (Santa Cruz) using ChIP kit (Cell Signaling Technology) according to the manufacturer’s protocol. Immunoprecipitated DNA released from the crosslinked proteins was quantitated with real-time PCR using the primers ( Supplementary Table 3 ) and was normalized to input DNA. Statistical analyses Statistical analysis was performed using analysis tools on the VassarStats Statistical Computation site ( http://vassarstats.net/ ) and Excel. Data were analysed using the parametric unpaired Student t -test, or two-way analysis of variance test for CIA scoring. How to cite this article: Yoon, J.-H. et al . Phosphorylation status determines the opposing functions of Smad2/Smad3 as STAT3 cofactors in T H 17 differentiation. Nat. Commun . 6:7600 doi: 10.1038/ncomms8600 (2015).